Microbe-dependent CD11b+IgA+plasma cells mediate robust early-phase intestinal IgA responses in mice Intestinal plasma cells predominantly produce immunoglobulin (Ig) A, however, their functional diversity remains poorly characterized. Here we show that murine intestinal IgA plasma cells can be newly classified into two populations on the basis of CD11b expression, which cannot be discriminated by currently known criteria such as general plasma cell markers, B cell origin and T cell dependence. CD11b + IgA + plasma cells require the lymphoid structure of Peyer’s patches, produce more IgA than CD11b − IgA + plasma cells, proliferate vigorously, and require microbial stimulation and IL-10 for their development and maintenance. These features allow CD11b + IgA + plasma cells to mediate early-phase antigen-specific intestinal IgA responses induced by oral immunization with protein antigen. These findings reveal the functional diversity of IgA + plasma cells in the murine intestine. Immunoglobulin (Ig) A is an antibody found predominantly in the intestinal lumen, where it protects the host against pathogenic infections [1] , [2] . It also has an important role in the creation and maintenance of immunological homoeostasis by shaping homeostatic communities of commensal bacteria [3] , [4] , [5] . Indeed, some patients with IgA deficiency show marked susceptibility to infections with pathogens such as Giardia lamblia , Campylobacter , Clostridium , Salmonella and rotavirus; they also have increased incidences of intestinal immune diseases such as coeliac disease and inflammatory bowel diseases [6] . Peyer’s patches (PPs) are the major sites for the initiation of antigen-specific intestinal IgA production, mainly in a T cell-dependent manner [7] . Intestinal IgA also originates from B1 cells. B1 cells differ from B2 cells in terms of origin, surface markers (for examples, B220, IgM, IgD, CD5, CD11b and CD23), growth properties and V H repertoire [8] , [9] , [10] . B1 cells are predominantly present in the peritoneal cavity (PerC) and traffic into the intestinal compartment for the production of IgA against T cell-independent antigens such as DNA and phosphatidylcholine [11] . T cell independent antigen-specific IgA responses are also initiated in the isolated lymphoid follicles (ILFs), which are small clusters of B2 cells in the intestine [12] . Upon Ig class switching from μ to α, IgA + B cells acquire the expression of type 1 sphingosine-1-phosphate receptor, CCR9 and α4β7 integrin, allowing them to migrate out from the PPs or PerC and traffic to the intestinal lamina propria (iLP) [11] , [13] , [14] . In the iLP, they further differentiate into IgA-secreting plasma cells (PCs) under the influence of terminal differentiation factors (for example, IL-6) [15] . As these locally produced IgA antibodies are continuously transported and secreted by epithelial cells as a form of secretory IgA into the intestinal lumen, stably high levels of IgA production are required for the maintenance of sufficient amounts of IgA; this production is determined by the generation, survival and function of IgA PCs. Several lines of evidence have demonstrated that the function and survival of PCs in the systemic compartments (for example, spleen and bone marrow (BM)) are not only determined by intrinsic factors but are regulated by the presence of environmental niches [16] . As with systemic PCs, differentiation of IgA PCs in the iLP is regulated by exogenous factors such as IgA-enhancing cytokines (for example, interleukin (IL)-5, IL-6, IL-10, IL-15, a proliferation-inducing ligand (APRIL) and B cell activating factor (BAFF)) [7] , [15] . In addition, microbial stimulation is required for the full effects of intestinal IgA. Indeed, germ-free (GF) mice have decreased intestinal IgA responses with immature structures of PPs and ILFs [17] , [18] . Previous studies in monoassociated GF mice have indicated that only a small proportion of the total amount of intestinal IgA is reactive to monoassociated bacteria; microbe-dependent IgA production is therefore mediated by polyclonal stimulation through innate immune receptors such as toll-like receptors, rather than through B cell receptors specific for microbial antigens [19] , [20] . Accumulating evidence has revealed the molecular and cellular pathways of IgA production mediated by innate immunity, including the involvement of myeloid differentiation primary response gene 88 (MyD88) in the regulation of tumour necrosis factor/inducible nitric oxide synthase-producing DCs in the iLP [21] and follicular DCs in the PPs [22] . However, the effects of microbial stimulation on the regulation of differentiated IgA + PCs remain to be investigated. Here, we identified unique microbe-dependent subsets of IgA + PCs, which add a new level of complexity to the intestinal IgA system of mice. Microbe dependency of intestinal IgA + cells To examine the immunological elements of intestinal IgA production associated with commensal bacteria, we initially compared the IgA + cells of specific pathogen-free (SPF) and GF mice. Flow cytometric analysis showed that CD11b + IgA + cells accounted for about 30% of IgA + cells, and we found a lack of CD11b + IgA + cells in the iLP of GF mice ( Fig. 1a ). Similarly, the numbers of intestinal CD11b + IgA + cells were reduced in both antibiotic-treated SPF mice and MyD88 KO mice ( Fig. 1b–d ). Immunohistological analysis indicated that CD11b + IgA + cells were dispersed throughout the iLP of wild-type (WT) mice ( Fig. 1d ), although their frequency appeared lower than expected from the flow cytometric data, probably because of difference in methodological sensitivity. These findings collectively suggest that CD11b + IgA + cells are unique subset that requires MyD88-dependent microbial stimulation for its development and maintenance. 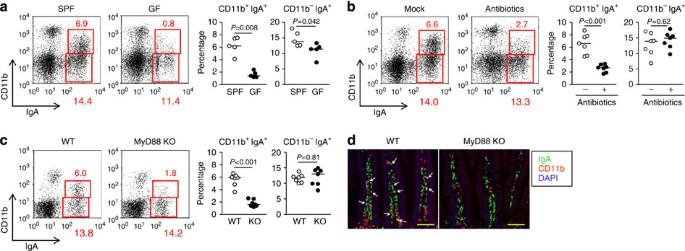Figure 1: Intestinal CD11b+IgA+cells require microbial stimulation. (a–c) Mononuclear cells were isolated from the small intestines of SPF or GF mice (a), mock- or antibiotic-treated SPF mice (b), or MyD88 WT or knockout (KO) mice (c) for analysis of IgA and CD11b expression by flow cytometry. Graphs show data from individual mice, and bars indicate median. Statistical analyses were performed with Mann–Whitney’sU-test. (d) Specimens of small intestinal tissues of WT and MyD88 KO mice were stained for IgA and CD11b, and counterstained with 4′,6-diamidino-2-phenylindole. Data are representative of three independent experiments. Scale bars, 50 μm. Figure 1: Intestinal CD11b + IgA + cells require microbial stimulation. ( a – c ) Mononuclear cells were isolated from the small intestines of SPF or GF mice ( a ), mock- or antibiotic-treated SPF mice ( b ), or MyD88 WT or knockout (KO) mice ( c ) for analysis of IgA and CD11b expression by flow cytometry. Graphs show data from individual mice, and bars indicate median. Statistical analyses were performed with Mann–Whitney’s U -test. ( d ) Specimens of small intestinal tissues of WT and MyD88 KO mice were stained for IgA and CD11b, and counterstained with 4′,6-diamidino-2-phenylindole. Data are representative of three independent experiments. Scale bars, 50 μm. Full size image Intestinal CD11b + IgA + cells are PCs We next aimed to characterize the CD11b + and CD11b − IgA + cells in the iLP. In addition to a gating strategy to exclude the possibility that the CD11b + IgA + cells detected by flow cytometry were doublets ( Supplementary Fig. S1 ), we further performed a cytospin analysis and confirmed that both CD11b + and CD11b − IgA + cells had homogeneous morphology that was the same as that of PCs (for example, large irregular nuclei with prominent nucleoli), whereas CD11b hi IgA – cells were composed of different kinds of cells, including eosinophils and macrophages ( Fig. 2a ). We also confirmed that both CD11b + and CD11b − IgA + cells did not express markers for macrophages (F4/80), DCs (CD11c) or eosinophils (CCR3) ( Fig. 2b ). Thus, CD11b + IgA + cells are neither doublets nor myeloid cells decorated by bound IgA on their surfaces. 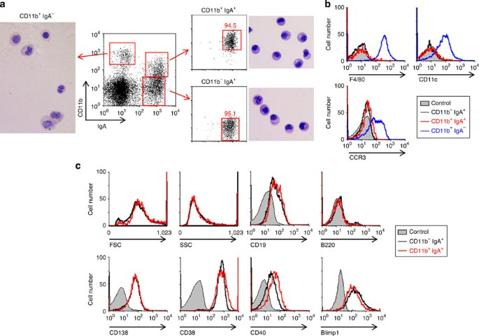Figure 2: Both CD11b+and CD11b−IgA+cells in the intestine are categorized as plasma cells. (a) Cells were purified by cell sorting from the iLP, and their morphology was examined by haematoxylin and eosin staining after cytospin. Data are representative of three independent experiments. (b) Cells were isolated from the iLP for the analysis of F4/80, CD11c and CCR3 expression on CD11b−IgA+, CD11b+IgA+and CD11b+IgA−cells. Grey indicates isotype control. Similar results were obtained from three separate experiments. (c) Cells were isolated from the iLP for comparisons between CD11b+and CD11b−IgA+cells in terms of cell size (FSC) and density (SSC), and expression of CD19, B220, CD138, CD38, CD40 and Blimp1. Grey indicates isotype control. Similar results were obtained from five separate experiments. Figure 2: Both CD11b + and CD11b − IgA + cells in the intestine are categorized as plasma cells. ( a ) Cells were purified by cell sorting from the iLP, and their morphology was examined by haematoxylin and eosin staining after cytospin. Data are representative of three independent experiments. ( b ) Cells were isolated from the iLP for the analysis of F4/80, CD11c and CCR3 expression on CD11b − IgA + , CD11b + IgA + and CD11b + IgA − cells. Grey indicates isotype control. Similar results were obtained from three separate experiments. ( c ) Cells were isolated from the iLP for comparisons between CD11b + and CD11b − IgA + cells in terms of cell size (FSC) and density (SSC), and expression of CD19, B220, CD138, CD38, CD40 and Blimp1. Grey indicates isotype control. Similar results were obtained from five separate experiments. Full size image CD11b + and CD11b − IgA + cells were identical in cell size and density, as determined by forward scatter (FSC) and side scatter (SSC), respectively, and by their surface expression patterns (CD19 int , B220 – , CD138 + , CD38 hi and CD40 int ) ( Fig. 2c ). Although PCs in the systemic compartments (for example, the spleen) generally express little or no surface immunogloblin [23] , we previously confirmed that CD38 + CD138 + cells in the iLP express IgA both on the cell surface and in the intracellular compartment ( Supplementary Fig. S2 ) [13] . These findings indicated that both CD11b + and CD11b − IgA + cells could be classically categorized as PCs. This view was further supported by our finding that both populations expressed equal levels of Blimp1, a master transcription factor for PCs ( Fig. 2c ) [23] . The phenotypes of IgA + cells in the iLP differed from those of IgA + cells in the spleen. Splenic CD11b − IgA + cells exclusively had a memory phenotype (that is, B220 + , CD138 – , CD38 int and CD40 hi ), whereas splenic CD11b + IgA + cells contained almost equal amounts of B220 + CD138 – CD38 int CD40 hi memory cells and B220 – CD138 + CD38 hi CD40 low PCs ( Supplementary Fig. S3 ). These results indicated that CD11b + IgA + cells in the iLP were unique PCs that had an immunologically different status from splenic CD11b + IgA + cells. Intestinal CD11b + IgA + PCs require PP lymphoid structure CD11b + IgA + PCs expressed CD18 ( Supplementary Fig. S4 ), which associates with CD11b and acts as a ligand for intercellular adhesion molecule-1 (ICAM-1) [24] . As ICAM-1 is an endothelial adhesion molecule that regulates cell trafficking [24] , [25] , we considered that CD11b + IgA + PCs were recent emigrants from IgA-inductive tissues (for example, PPs and PerC) and had migrated into the iLP. To test this possibility, we employed FTY720 to inhibit the trafficking of IgA-committed B cells from PPs and PerC into the iLP. As we previously reported [11] , [13] , FTY720 treatment reduced the numbers of intestinal IgA + PCs, but the effect was not specific to CD11b + IgA + PCs ( Fig. 3a ). These data suggested that CD11b + IgA + PCs were not recent emigrants from IgA inductive tissues (for example, PPs and PerC). 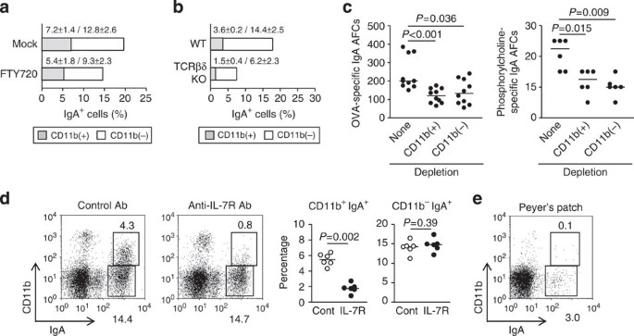Figure 3: CD11b+IgA+cells require the lymphoid structure of Peyer’s patches. (a) Mice were treated with FTY720 every day for 5 days. The day after the final treatment, the proportions of CD11b+and CD11b−IgA+cells were measured by flow cytometry. Data are presented as means±s.d. from four mice. Similar results were obtained from three separate experiments. (b) Proportions of CD11b+and CD11b−IgA+cells in the iLP of WT and TCRβδ KO mice were measured by flow cytometry. Data are presented as means±s.d. from four mice. Similar results were obtained from three separate experiments. (c) After three oral immunizations with OVA plus cholera toxin, cells were isolated from the iLP and used in an ELISPOT assay to enumerate OVA-specific IgA AFCs. In some groups of mice, CD11b+or CD11b−IgA+cells were depleted by cell sorting before application of ELISPOT assay. Phosphorylcholine-specific IgA AFCs were measured. Graphs show data from individual mice, and bars indicate median. Statistical analyses were performed with Mann–Whitney’sU-test. (d) Mononuclear cells were isolated from the iLP of Peyer’s patch (PP)-normal (control Ab) and -null (anti-IL-7Rα Ab) mice for analysis of IgA and CD11b expression by flow cytometry. Graphs show data from individual mice. Statistical analyses were performed with Mann–Whitney’sU-test. (e) Mononuclear cells were isolated from PPs for analysis of CD11b+and CD11b−IgA+cells by flow cytometry. Similar results were obtained from three separate experiments. Figure 3: CD11b + IgA + cells require the lymphoid structure of Peyer’s patches. ( a ) Mice were treated with FTY720 every day for 5 days. The day after the final treatment, the proportions of CD11b + and CD11b − IgA + cells were measured by flow cytometry. Data are presented as means±s.d. from four mice. Similar results were obtained from three separate experiments. ( b ) Proportions of CD11b + and CD11b − IgA + cells in the iLP of WT and TCRβδ KO mice were measured by flow cytometry. Data are presented as means±s.d. from four mice. Similar results were obtained from three separate experiments. ( c ) After three oral immunizations with OVA plus cholera toxin, cells were isolated from the iLP and used in an ELISPOT assay to enumerate OVA-specific IgA AFCs. In some groups of mice, CD11b + or CD11b − IgA + cells were depleted by cell sorting before application of ELISPOT assay. Phosphorylcholine-specific IgA AFCs were measured. Graphs show data from individual mice, and bars indicate median. Statistical analyses were performed with Mann–Whitney’s U -test. ( d ) Mononuclear cells were isolated from the iLP of Peyer’s patch (PP)-normal (control Ab) and -null (anti-IL-7Rα Ab) mice for analysis of IgA and CD11b expression by flow cytometry. Graphs show data from individual mice. Statistical analyses were performed with Mann–Whitney’s U -test. ( e ) Mononuclear cells were isolated from PPs for analysis of CD11b + and CD11b − IgA + cells by flow cytometry. Similar results were obtained from three separate experiments. Full size image The second possibility was that CD11b + IgA + PCs originated from B1 cells, because CD11b is a marker of peritoneal B1 cells [26] . To test this possibility, peritoneal CD11b + B1 cells were purified and adoptively transferred into severe combined immunodeficiency mice. As we reported previously [11] , adoptively transferred CD11b + B1 cells migrated into the intestine, where they differentiated into IgA + PCs. Although we transferred B cells expressing CD11b, they lost their CD11b expression in the iLP ( Supplementary Fig. S5 ). Although only a few cells were detected in the iLP under these experimental conditions, CD11b expression was likely to be reversible on B cells and was thus not to be a marker of PCs originating from peritoneal CD11b + B1 cells. As a third possibility for discriminating between CD11b + and CD11b − IgA + PCs, we examined the T cell dependency of their differentiation and IgA production. For this, we employed TCRβδ mice. Although TCRβ δ mice had decreased levels of intestinal IgA + cells, the ratio between CD11b + and CD11b − IgA + PCs did not differ between the WT mice and the TCRβ δ mice ( Fig. 3b ). We also examined the production of IgA against T cell dependent and T cell independent antigens by CD11b + and CD11b − IgA + PCs. For the analysis of T cell dependent antigen, mice were orally immunized with ovalbumin (OVA) plus cholera toxin (CT). Following three oral immunizations, substantial amounts of OVA-specific IgA antibody-forming cells (AFCs) were detected in the iLP by enzyme-linked immunosorbent spot (ELISPOT) assay; this production was reduced by almost 50% when either the CD11b + IgA + or the CD11b − IgA + cells were removed before the ELISPOT assay ( Fig. 3c ). Similar results were obtained when we enumerated IgA AFCs against phosphorylcholine, a typical TI antigen, induced by commensal bacteria ( Fig. 3c ) [27] . These results collectively suggested that both CD11b + IgA + and CD11b − IgA + cells almost equally included IgA AFCs producing IgA antibodies specific for T cell dependent and T cell independent antigens. Next, to examine the involvement of PPs, we established PP-null mice by in utero treatment with anti-IL-7Rα antibody [28] and found that PP-null mice had reduced numbers of CD11b + IgA + PCs in the iLP ( Fig. 3d ). In addition, CD11b was not expressed on IgA + B cells in the PPs ( Fig. 3e ). We treated mice with anti-IL-7Rα antibody only once in utero and confirmed that it did not affect the ILFs [28] . Although it is still possible that CD11b + IgA + PCs specifically require IL-7, the most plausible conclusion based on our current findings is that CD11b + IgA + B cells require the lymphoid structure of PPs, and CD11b − IgA + B cells acquire CD11b expression in the iLP. As in antibiotic-treated and MyD88 KO mice ( Fig. 1 ), the numbers of CD11b − IgA + PCs changed little in PP-null mice ( Fig. 3d ), suggesting that it is unlikely that CD11b + IgA + PCs differentiate back into CD11b − IgA + cells in the iLP. This view is further supported by the results of in vitro analysis. When purified CD11b + and CD11b − IgA + PCs were separately cultured with different kinds of stimulants (for example, phorbol 12-myristate 13-acetate plus ionomycin, or lipopolysaccharide) little change was noted in CD11b expression ( Supplementary Fig. S6 ). Although the origin of these cells remains to be firmly established, it is plausible that CD11b + IgA + PCs act as a separate lineage once they differentiate in the iLP. High proliferation activity of CD11b + IgA + PCs We next performed a gene microarray analysis to assess the uniqueness of CD11b + IgA + PCs in the iLP. Gene ontology enrichment score computation analysis showed that the activity of cell-cycle-associated pathways was higher in CD11b + IgA + PCs than in CD11b − IgA + PCs ( Supplementary Table S1 ). Consistent with this finding, higher expression of cell-cycle-associated genes was noted in CD11b + IgA + PCs than in CD11b − IgA + PCs; these genes included members of the cell division cycle family ( Fig. 4a and Supplementary Table S2 ). In line with this, these cells expressed higher levels of the proliferation marker Ki67 than did CD11b − IgA + PCs ( Fig. 4a and Supplementary Table S2 ). Additionally, CD11b + IgA + PCs showed greater uptake of bromodeoxyuridine (BrdU) than did CD11b − IgA + PCs ( Fig. 4b ). CD11b + IgA + PCs were preferentially removed by treatment with cyclophosphamide (CPM), which selectively targets proliferating cells ( Fig. 4c ). These data collectively suggested that CD11b + IgA + PCs possessed greater proliferating activity than did CD11b − IgA + PCs in the iLP. 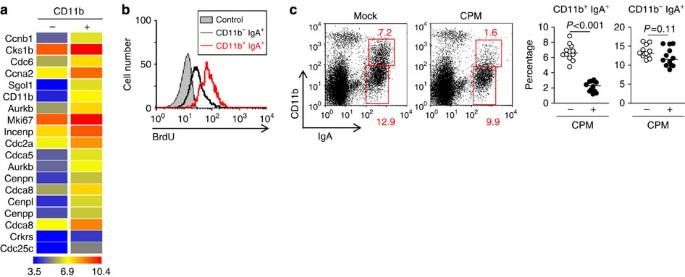Figure 4: CD11b+IgA+cells are proliferating cells. (a) mRNA was purified from small intestinal CD11b+and CD11b−IgA+cells and used for microarray analysis. Data related to the cell cycle and proliferation are shown. Data are representative of two independent experiments. (b) Mice were treated with BrdU, and uptake of BrdU by CD11b+and CD11b−IgA+cells was determined by flow cytometry. Data are representative of four independent experiments. (c) Cells were isolated from the intestinal lamina propria of mice receiving CPM to analyse CD11b+IgA+cells. Similar results were obtained from four separate experiments. Graphs show data from individual mice. Statistical analyses were performed with Mann–Whitney’sU-test. Figure 4: CD11b + IgA + cells are proliferating cells. ( a ) mRNA was purified from small intestinal CD11b + and CD11b − IgA + cells and used for microarray analysis. Data related to the cell cycle and proliferation are shown. Data are representative of two independent experiments. ( b ) Mice were treated with BrdU, and uptake of BrdU by CD11b + and CD11b − IgA + cells was determined by flow cytometry. Data are representative of four independent experiments. ( c ) Cells were isolated from the intestinal lamina propria of mice receiving CPM to analyse CD11b + IgA + cells. Similar results were obtained from four separate experiments. Graphs show data from individual mice. Statistical analyses were performed with Mann–Whitney’s U -test. Full size image Microarray analysis further identified CD150 (also known as signalling lymphocytic activation molecule family member 1, SLAMF1) [29] , β1 integrin and CD168 (also known as hyaluronan-mediated motility receptor) [30] as possible candidates uniquely expressed on CD11b + IgA + PCs ( Supplementary Table S3 ). Flow cytometric analysis confirmed that CD11b + IgA + PCs expressed higher levels of CD150 than did CD11b − IgA + PCs, whereas CD11b + IgA + and CD11b − IgA + PCs identically expressed β1 integrin and no CD168 ( Supplementary Fig. S7 ). IL-10 is essential for intestinal CD11b + IgA + cells We next aimed to identify key molecules for inducing and maintaining CD11b + IgA + PCs in the iLP. As CD11b + IgA + PC numbers were reduced in MyD88 mice ( Fig. 1c ), and MyD88 is expressed in not only hematopoietic cells, including B cells, but also non-hematopoietic cells, including epithelial cells [31] , we performed BM chimeric experiments to determine whether MyD88 in non-hematopoietic cells, hematopoietic cells, or both, was required for the generation of CD11b + IgA + cells. Similar levels of CD11b + IgA + cells were observed in irradiated WT mice receiving WT or MyD88 BM cells and in irradiated MyD88 mice receiving WT BM cells ( Supplementary Fig. S8 ), suggesting that MyD88-dependent molecules commonly expressed in both non-hematopoietic and hematopoietic cells are involved in the microbe-dependent induction of CD11b + IgA + PCs. We then examined the involvement of cytokines known to enhance IgA responses. Among several IgA-enhancing cytokines (for example, IL-5, IL-6, IL-10 and APRIL/BAFF) [7] , [15] , we found that neutralization of IL-10 resulted in preferential reduction in CD11b + IgA + PCs, whereas blocking of other cytokines induced a reduction in IgA + cell numbers regardless of CD11b expression ( Fig. 5a ). Additionally, CD11b + IgA + cell numbers were preferentially reduced in IL-10 KO mice ( Fig. 5b ). As normal differentiation into IgA + B cells was observed in the PPs and PerC of IL-10 KO mice ( Supplementary Fig. S9 ), it is plausible that IL-10 targets the maintenance of CD11b + IgA + cells in the iLP, but not the induction of IgA + cells in inductive tissues such as PPs and PerC. 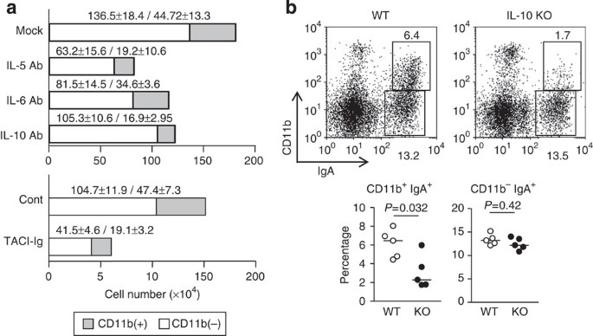Figure 5: Role of IL-10 in the maintenance of CD11b+IgA+cells in the iLP. (a) Mice were treated with antibodies to block IL-5, IL-6, IL-10 or antagonistic TACI-immunoglobulin (TACI-Ig) fusion protein. Mononuclear cells were isolated from the iLP and used for analysis of CD11b+and CD11b−IgA+cells by flow cytometry. Data are presented as means±s.d. (n=4). (b) Mononuclear cells were isolated from the iLP of WT or IL-10 KO mice for analysis of IgA and CD11b expression by flow cytometry. Graphs show data from individual mice. Statistical analyses were performed with Mann–Whitney’sU-test. Figure 5: Role of IL-10 in the maintenance of CD11b + IgA + cells in the iLP. ( a ) Mice were treated with antibodies to block IL-5, IL-6, IL-10 or antagonistic TACI-immunoglobulin (TACI-Ig) fusion protein. Mononuclear cells were isolated from the iLP and used for analysis of CD11b + and CD11b − IgA + cells by flow cytometry. Data are presented as means±s.d. ( n =4). ( b ) Mononuclear cells were isolated from the iLP of WT or IL-10 KO mice for analysis of IgA and CD11b expression by flow cytometry. Graphs show data from individual mice. Statistical analyses were performed with Mann–Whitney’s U -test. Full size image Early-phase robust IgA responses by proliferating IgA + PCs To examine the immunological importance of proliferating IgA + PCs present mainly in CD11b + IgA + PCs, mice were orally immunized with OVA plus CT. In this assay, one group received CPM treatment during immunization and the second group received CPM treatment 4 days after the final immunization ( Fig. 6a ). Because of the high cell-proliferation activity, CPM treatment during oral immunization resulted in efficient killing of peanut agglutinin (PNA hi ) B220 + GC B cells and thus a reduction in the numbers of IgA + IgM – plasmablasts in the PPs ( Supplementary Fig. S10 ). Thus, treatment with CPM during oral immunization led to an ~90% reduction in the numbers of OVA-specific IgA AFCs ( Fig. 6b ); this was associated with almost complete disappearance of faecal IgA produced against OVA ( Fig. 6c ). On the other hand, when mice were treated with CPM 4 days after the final immunization to remove proliferating cells mainly present in CD11b + IgA + cells in the iLP, the reduction in numbers of OVA-specific IgA AFCs in the iLP was only about 50% ( Fig. 6b ). This finding was consistent with our current finding that CD11b + IgA + PCs accounted for half the number of OVA-specific IgA AFCs ( Fig. 3c ). Thus, CPM treatment after the last immunization preferentially depleted CD11b + IgA + cells, with little influence on CD11b − IgA + cells. Of note, these mice showed ~90% reduction in OVA-specific IgA content in the faeces compared with mice not treated with CPM ( Fig. 6c ). We also confirmed that CPM treatment 4 days after final immunization induced a reduction in the production of IgA specific to the B subunit of CT (that is, CTB), which was associated with the halving of the abundance of CTB-specific IgA AFCs in the intestine ( Fig. 6d ). Like OVA-specific IgA responses ( Figs. 3c and 6b ), similar levels of reduction of CTB-specific IgA AFCs were noted when CD11b + IgA + cells were depleted before ELISPOT assay ( Fig. 6e ). These mice showed reduced resistance to oral challenge with CT and developed watery diarrhoea ( Fig. 6f and Supplementary Fig. S11 ). 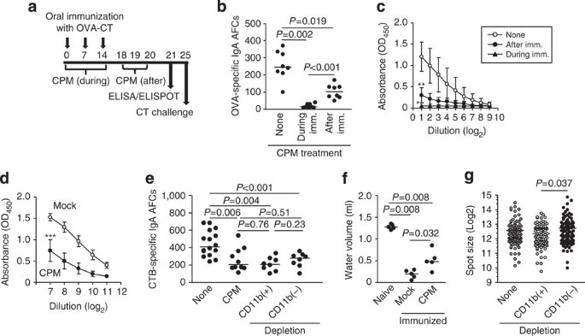Figure 6: Proliferating IgA+cells mediate early-phase IgA responses to oral antigen. (a) Experimental schedule for oral immunization and CPM treatment. Mice were orally immunized with OVA plus CT on days 0, 7 and 14. One group received CPM during oral immunization (days 0, 7 and 14) and another received CPM after the last immunization (days 18, 19 and 20). (b,c) One week after the final immunization (day 21), mononuclear cells were isolated from the iLP to quantify OVA-specific IgA-forming cells by ELISPOT (b). Simultaneously, faeces (c,d) were collected and were used for the detection of the (c) OVA-or (d) B subunit of CT (CTB)-specific IgA by enzyme-linked immunosorbent assay. Data are from individual mice and bars indicate median (b) and represent means±s.d. (n=10) from two separate experiments (c,d). *P<0.001, **P<0.01, ***P<0.05 (two tailed unpairedt-test). (e) Mononuclear cells were isolated from the iLP of mock- or CPM-treated mice 1 week after the final immunization to quantify CTB-specific IgA-forming cells by ELISPOT. In some groups of mock-treated mice, CD11b+or CD11b−IgA+cells were depleted by cell sorting before application of ELISPOT assay. Graphs show data from individual mice, and bars indicate median. (f) On day 21, mice were orally challenged with 100 μg CT. After 15 h, the volume of intestinal fluid was measured. Graphs show data from individual mice, and bars indicate median. Similar results were obtained from two separate experiments. (g) Spot sizes of CTB-specific IgA AFCs were measured by Zeiss KS ELISPOT software. Graphs show data from individual mice, and bars indicate median. Statistical analyses were performed with Mann–Whitney’sU-test (e–g). Figure 6: Proliferating IgA + cells mediate early-phase IgA responses to oral antigen. ( a ) Experimental schedule for oral immunization and CPM treatment. Mice were orally immunized with OVA plus CT on days 0, 7 and 14. One group received CPM during oral immunization (days 0, 7 and 14) and another received CPM after the last immunization (days 18, 19 and 20). ( b , c ) One week after the final immunization (day 21), mononuclear cells were isolated from the iLP to quantify OVA-specific IgA-forming cells by ELISPOT ( b ). Simultaneously, faeces ( c , d ) were collected and were used for the detection of the ( c ) OVA-or ( d ) B subunit of CT (CTB)-specific IgA by enzyme-linked immunosorbent assay. Data are from individual mice and bars indicate median ( b ) and represent means±s.d. ( n =10) from two separate experiments ( c , d ). * P <0.001, ** P <0.01, *** P <0.05 (two tailed unpaired t -test). ( e ) Mononuclear cells were isolated from the iLP of mock- or CPM-treated mice 1 week after the final immunization to quantify CTB-specific IgA-forming cells by ELISPOT. In some groups of mock-treated mice, CD11b + or CD11b − IgA + cells were depleted by cell sorting before application of ELISPOT assay. Graphs show data from individual mice, and bars indicate median. ( f ) On day 21, mice were orally challenged with 100 μg CT. After 15 h, the volume of intestinal fluid was measured. Graphs show data from individual mice, and bars indicate median. Similar results were obtained from two separate experiments. ( g ) Spot sizes of CTB-specific IgA AFCs were measured by Zeiss KS ELISPOT software. Graphs show data from individual mice, and bars indicate median. Statistical analyses were performed with Mann–Whitney’s U -test ( e – g ). Full size image These findings led us to hypothesize that CD11b + IgA + PCs are capable of producing more IgA than are CD11b − IgA + PCs. To test this hypothesis, we measured the size of each spot in CTB-specific IgA AFCs in an ELISPOT assay. The cells in the CD11b + IgA + cell-enriched fraction (depletion of CD11b − IgA + cells) were bigger than those in the CD11b − IgA + cell-enriched fraction (depletion of CD11b + IgA + cells) ( Fig. 6g ). Furthermore, an adoptive transfer experiment demonstrated higher intestinal IgA production in severe combined immunodeficiency mice receiving CD11b + IgA + PCs than in those receiving CD11b − IgA + PCs ( Supplementary Fig. S12 ), presumably because of both high IgA production and proliferating activity of CD11b + IgA + PCs. Although some possibilities (for example, proliferation and CD11b expression of IgA + cells might be changed during immunization) cannot be excluded, it is plausible that the actual production of IgA secreted into the intestinal lumen was derived mainly from CD11b + IgA + PCs in the early phase of the IgA response against orally immunized antigen. PCs could secrete antibodies to provide antigen-specific humoral immune responses in both systemic and mucosal tissues. Here, we demonstrated that intestinal IgA + PCs in mice could be categorized into two populations on the basis of CD11b expression. CD11b is an integrin αM that non-covalently associates with CD18 to form αMβ2 integrin (Mac-1) and binds to ICAM-1 (ref. 24 ). We therefore expected that CD11b + IgA + PCs were newly migrating cells whose migration was mediated by endothelial cells expressing ICAM-1, but in fact they were not. We also found no uptake of opsonized bacteria in either CD11b + or CD11b − IgA + cells ( Supplementary Table S4 and Supplementary Fig. S13a ), although CD11b is a receptor for complement (iC3b) [24] . In addition, unlike in human CD11b + B cells, which stimulate T cells strongly [32] , major histocompatibility complex (MHC) class II (I-A d ) and costimulatory molecules (for example, CD80) were identically expressed on both CD11b + and CD11b − IgA + cells ( Supplementary Table S4 and Supplementary Fig. S13b ). A similar subset of CD11b + IgA + cells was observed in the systemic murine compartments (for example, spleen), but the immunological characteristics of these cells differed from those of the cells in the intestine. Indeed, intestinal CD11b + IgA + cells consisted exclusively of PCs, but not memory B cells, whereas splenic CD11b + IgA + cells included both PCs and memory B cells. We further found that CD11b could not be used as a marker of B1 cells in the intestine. Our current findings show for the first time that CD11b could be a specific marker for discriminating IgA + PCs that require microbial stimulation and IL-10, and presumably contribute to the early phase of the intestinal IgA response in mice. We have identified unique CD11b + IgA + PCs in mice; the next question is whether or not the same population of IgA + PCs exists in humans. Our preliminary experiments have shown that no human intestinal IgA + cells express CD11b, but that some IgA + cells express Ki67, a marker of proliferating cells (unpublished data). One possible explanation for this difference between human and mice is difference in the composition of commensal bacteria. In this regard, we examined the involvement of segmented filamentous bacteria (SFB), which are a known major IgA stimulus in mice, but has not yet been confirmed as part of the human microbiota [19] . As expected, SFB stimulated IgA production following colonization of SFB-deficient C57BL/6 mice from the Jackson laboratory (JAX mice) with bacterial suspensions from SFB-monoassociated mice (JAX+SFB mice) [33] ; however, we found that CD11b is expressed on IgA + cells independently of SFB colonization ( Supplementary Fig. S14 ). It is possible that other commensal bacteria such as Lactobacillus (abundant in mice) and Bifidobacterium (abundant in human) are responsible for the species-specific expression of CD11b on IgA + cells. It is important to recognize the differences between the mouse and human immune systems, but it is obvious that proliferating IgA + cells are present in the iLP of both mouse and human. The immunological function of human proliferating IgA + cells in the intestine will therefore be the subject of our next study. In the initial step of the antibody response to T cell dependent antigens, B cells are activated by antigens and form GCs in the lymph nodes [7] . As depleting antigen-specific GC B cells by CPM treatment during oral immunization resulted in complete loss of the IgA response to orally immunized antigen, it is likely that both CD11b + and CD11b − IgA + PCs against T cell dependent antigen are derived from GC B cells. We also found that depletion of proliferating CD11b + IgA + PCs by CPM treatment after final immunization led to a decrease in the early-phase IgA response, although it is possible that proliferation activity and/or CD11b expression on IgA + cells might be wobble during immunization. Our in vivo findings indicated that the reduction in CD11b + IgA + PC numbers in MyD88 KO, IL-10 KO and PP-null mice did not affect the numbers of CD11b − IgA + PCs ( Figs 1c ). These findings, together with our in vitro data ( Supplementary Fig. S6 ), indicate that it is likely that CD11b + IgA + PCs act as a separate lineage once they differentiate in the iLP. Proliferating CD11b + IgA + PCs required microbial stimulation in the intestine. As proliferation is one of the characteristics of plasmablasts, it was possible that CD11b + IgA + cells have been recently committed to the PC fate. Notably, intestinal IgA + cells expressed MHC class II molecules; this expression is one of the unique characteristics of plasmablasts. Therefore, it is likely that intestinal IgA + PCs partly retain their plasmablast features. However, our findings indicated that CD11b + and CD11b − IgA + cells expressed identical levels of Blimp-1 and MHC class II. In addition, similar reduction was noted in CD11b + and CD11b − IgA + cells when cell trafficking from IgA inductive tissues (for example, PPs and the PerC) into the iLP was inhibited by treatment with FTY720. Thus, our findings suggest that CD11b + IgA + cells uniquely exhibit high proliferating and IgA-producing activity, although their other immunological features as PCs are similar to those of CD11b − IgA + PCs. Proliferating CD138 + PCs have been detected in the spleens of NZB/W mice with signs of systemic lupus erythematosus, but not in naive mice [34] . In contrast, the number of non-proliferating CD138 + PCs is unchanged in the intestines of GF mice, as it is in the spleens of NZB/W mice [34] . These findings suggest that MyD88-dependent homeostatic stimulation of commensal bacteria determines the fate of proliferating CD11b + IgA + CD138 + PCs in the intestine. Several lines of evidence have revealed the cellular and molecular mechanisms of microbe-dependent initiation of IgA responses. B cells express several toll-like receptors, and B cell-intrinsic MyD88-mediated signalling has been implicated in enhanced antibody production in some studies [35] , [36] . However, our current findings indicated that MyD88-mediated signalling in hematopoietic cells, including B cells, was not essential for intestinal CD11b + IgA + PC production. Additionally, we found IL-10 as a key molecule inducing CD11b + IgA + PC production. Previous studies have demonstrated that IL-10 promotes the proliferation of activated B cells and subsequent IgA production in vitro [37] , [38] , which are consistent with our current findings of high-level proliferation of, and IgA production by, CD11b + IgA + PCs. Thus, our current findings proved that IL-10 functions in IgA production in vivo and that CD11b + IgA + PCs are the main targets in this pathway. Despite these findings, our preliminary study demonstrated that treatment of CD11b + or CD11b − IgA + PCs with IL-10 alone did not induce their reciprocal differentiation into each other, and IL-10 KO mice with colitis possessed CD11b + IgA + PCs (J.K., unpublished data). Thus, IL-10 is redundant in some cases and additional factors are required for the maintenance of CD11b + IgA + PCs. Our current findings identified CD150 as a surface molecule that is highly expressed on CD11b + IgA + PCs. CD150 is a 70-kDa glycoprotein expressed on some B and T cells, thymocytes and macrophages [29] . Homophilic interaction of CD150 induces proliferation of, and antibody synthesis by, B cells [39] , and notably IL-10 synergistically enhances CD150-mediated B cell proliferation [39] . Thus, it is likely that, at least partly, IL-10 and CD150 determine the unique features (for example, proliferation and high IgA production) of CD11b + IgA + PCs in the iLP. In addition, accumulating evidence has revealed an important immunological function of stromal cells as survival niches for PCs in the BM [40] and intestine [41] , [42] . It is possible that complex immunological communications among commensal flora, epithelial and stromal cells, and the cells involved in innate and acquired immunity determine the differentiation and maintenance of IgA PCs in the intestine. Taken together, our results provide new insights into the nature of IgA + PCs in the murine intestine, and especially into the regulation of the early-phase IgA responses to intestinal antigens and requirement of microbe-dependent stimulation, IL-10, and the PP lymphoid structure. These findings add a new level of complexity to the intestinal IgA system of mice. Mice SPF and GF Balb/c mice were obtained from Japan CLEA (Tokyo, Japan). MyD88 KO mice, IL-10 mice (Balb/c background) and TCRβδ mice (C57/BL6 background) were maintained under SPF conditions at the Experimental Animal Facility, The Institute of Medical Science, The University of Tokyo, and WT littermates were used as controls. To deplete gut commensal bacteria, mice received broad-spectrum antibiotics, namely ampicillin (1 g l −1 ; Sigma-Aldrich, St Louis, MO), vancomycin (500 mg l −1 ; Shionogi, Osaka, Japan), neomycin sulphate (1 g l −1 ; Sigma-Aldrich) and metronidazole (1 g l −1 ; Sigma-Aldrich), in their drinking water for 4 weeks [43] . To establish BM chimeric mice, we injected γ-irradiated (960 rad, Gammacell 40, Atomic Energy of Canada Limited, Ontario, Canada) recipient mice with 5 × 10 6 BM cells through the tail vein and used them in experiments 8 weeks after injection. Under our experimental conditions, the reconstitution efficacy was about 90–95%. To obtain PP-null mice, pregnant BALB/c mice were injected intravenously and subcutaneously with 1 mg anti-IL-7Rα antibody (A7R34, BioLegend, San Diego, CA) at 14.5 days post coitus, as described previously [28] . We confirmed the disruption of organized PPs and the existence of ILFs in the offspring, as described previously [28] . To neutralize cytokines, mice were treated intraperitoneally with 250 μg of monoclonal antibodies specific for IL-5 (TRFK5), IL-6 receptor (D7715A7) or IL-10 (JES5.16E3) (BioLegend, San Diego, CA); control antibody (Rat IgG2b); or 100 μg of soluble TACI-Fc fusion protein (R&D Systems, Minneapolis, MN) every second day for 2 weeks [44] , [45] . For assessing the role of SFB, mice purchased from the Jackson laboratory were orally inoculated with bacterial suspensions obtained by homogenizing faecal pellets from SFB-monoassociated mice in water. SFB colonization was confirmed by quantitative PCR [33] and CD11b + IgA + cells were analysed in the small intestine 2 weeks post gavage by flow cytometry. All experiments followed the guidelines of the Animal Care and Use Committee, The University of Tokyo and Columbia University. Oral immunization Mice were given sodium bicarbonate solution to neutralize stomach acid [11] , [13] . Thirty minutes later, the mice were orally immunized with 1 mg OVA (Sigma-Aldrich) and 10 μg CT (List Biological Laboratories, Campbell, CA). This procedure was conducted on days 0, 7 and 14. In some groups, mice were intraperitoneally given CPM (35 mg kg −1 each time, Sigma-Aldrich). One week after the final immunization, faecal samples and mononuclear cells from the iLP were collected for enumeration of OVA-specific antibody responses by enzyme-linked immunosorbent assay and ELISPOT, respectively [13] . In vivo CT challenge was performed by oral challenge of naive or immunized mice with 100 μg of CT as previously described [46] . Cell isolation To isolate mononuclear cells from PPs, we stirred the tissues in RPMI-1640 medium containing 2% fetal calf serum plus 0.5 mg ml −1 collagenase (Wako, Osaka, Japan) [11] , [13] . To isolate mononuclear cells from the iLP, PPs were carefully removed and the remaining intestines including ILFs were opened longitudinally, washed with RPMI-1640, cut into 2-cm pieces and stirred for 20 min at 37 °C into RPMI-1640 containing 0.5 mM EDTA and 2% fetal calf serum to remove epithelial cells and intraepithelial lymphocytes [11] , [13] . The tissues were then stirred three times in 0.5 mg ml −1 collagenase for 20 min before undergoing discontinuous Percoll gradient centrifugation (40 and 75%). Peritoneal cells were obtained by peritoneal flushing with 8 ml ice-cold phosphate-buffered saline (PBS) [11] , [13] . Flow cytometry and cell sorting Mononuclear cells were preincubated with 10 μg ml −1 anti-CD16/32 antibody (BD Biosciences, San Diego, CA). They were then reacted with the following antibodies: Pacific blue-rat anti-mouse CD45R (B220) (RA3-6B2, 0.8 μg ml −1 ), phycoerythrin (PE)-rat anti-mouse CD11b (M1/70, 0.1 μg ml −1 ), PE-Cy7-hamster anti-mouse CD11c (HL3, 0.4 μg ml −1 ), PE-rat anti-mouse CD18 (C71/16, 0.8 μg ml −1 ), PE-rat anti-mouse CD19 (1D3, 0.8 μg ml −1 ), PE-rat anti-mouse CD38 (90, 0.13 μg ml −1 ), FITC-rat anti-mouse IgA (C10-3, 2 μg ml −1 ), PE-Cy7-rat anti-mouse IgM (R6-60.2, 1 μg ml −1 ), PE-anti-mouse I-A d (AMS-32.1, 0.4 μg ml −1 ), APC-Cy7-rat anti-mouse CD11b (M1/70, 1 μg ml −1 ), APC-Cy7-anti-mouse β1-integrin (HMβ1-1, 4 μg ml −1 ), APC-anti-mouse CD40 (3/23, 2 μg ml −1 ), Pacific blue-anti-mouse CD11b (M1/70, 1 μg ml −1 ), PE-Cy7-anti-mouse F4/80 (BM8, 0.4 μg ml −1 ) and biotin mouse anti-CD138 (281-2, 10 μg ml −1 ) (all antibodies from BD Biosciences) followed by incubation with streptavidin-APC (1 μg ml −1 , BD Biosciences), PE-anti-mouse CD150 (TC15-12F12.2, 0.1 μg ml −1 ), Alexa Fluor 647-anti-mouse CD80 (16-10A1, 1 μg ml −1 ) (BioLegend, San Diego, CA), anti-mouse CD267 (TACI) (8F10-3, 4 μg ml −1 ) (eBioscience, San Diego, CA), PE-mouse CCR3 (83101, 0.5 μg ml −1 ) (R&D Systems) or biotinylated anti-peanut agglutinin lectin (1 μg ml −1 , Vector Laboratories, Burlingame, CA), followed by staining with streptavidin PE (1 μg ml −1 , BD Biosciences). For staining for Blimp-1, cells were fixed and permeabilized with a Cytofix/Cytoperm kit (BD Biosciences) and stained with PE-conjugated anti-Blimp1 goat polyclonal IgG (0.4 μg ml −1 , Santa Cruz Biotechnology, Santa Cruz, CA). FSC-H and FSC-A discrimination was used to exclude doublet cells, and ViaProbe cell-viability solution (BD Biosciences) was used to discriminate between dead and living cells. To detect proliferating cells, mice received 1 mg BrdU intraperitoneally 24 h before analysis; the BrdU signal was detected with the manufacturer’s protocol (BD Biosciences). Concentration-matched isotype antibodies were used as negative controls. Flow-cytometric analysis and cell sorting were performed with FACSCanto II and FACSAria (BD Biosciences), respectively. We confirmed that cell purity was about 95% ( Fig. 2a ). Immunohistological analysis Intestines were fixed in 4% paraformaldehyde for 15 h at 4 °C, washed with PBS and treated sequentially in 10 and 20% sucrose for 12 h at 4 °C 13 . The tissues were embedded in OCT compound (Sakura Finetechnical Co., Tokyo, Japan). Cryostat sections (7 μm) were pre-blocked with anti-CD16 and CD32 antibody for 15 min at room temperature and stained for 15 h at 4 °C with FITC-rat anti-mouse IgA (C10-3, 2 μg ml −1 ) and biotin anti-mouse CD11b antibody (M1/70, 1 μg ml −1 ). This was followed by incubation with horseradish peroxidase (HRP)-conjugated streptavidin (Pierce, Rockford, IL) for 30 min at 4 °C and amplification of the fluorescent signal with Cy3-tyramide (TSA-Direct kit; PerkinElmer, Waltham, MA) [13] . We confirmed that no signal was detected when the specimens were stained with the concentration-matched isotype antibodies. They were then counterstained with 4′,6-diamidino-2-phenylindole (Sigma-Aldrich). Deconvoluted fluorescence images of specimens were obtained by fluorescence microscopy (BZ9000, Keyence, Osaka, Japan). Detection of antibody responses by enzyme-linked immunosorbent assay and ELISPOT To measure OVA- or CTB-specific IgA levels in faecal extracts, faeces were homogenized in PBS by vigorous vortexing [11] , [13] . After centrifugation of the extracts (9,000 g for 15 min) the supernatants were used as faecal extracts. Plates were coated with 1 mg ml −1 OVA or 2 μg ml −1 CTB in PBS; this was followed by blocking for 1 h at room temperature with 200 μl PBS containing 1% (w/v) bovine serum albumin. After extensive washing of the plates with PBS containing 0.05% Tween 20, serial sample dilutions were added for incubation overnight at 4 °C. Samples were then incubated for 1 h at room temperature with optimally diluted HRP-conjugated goat anti-mouse IgA (SouthernBiotech, Birmingham, AL). After sample washing, the colour reaction was developed at room temperature with 3,3′,5,5′-tetramethylbenzidine (Moss, Pasadena, MD) and terminated by adding 0.5 M HCl. The colour reaction was measured as the optical density (wavelength 450 nm). ELISPOT assay was used to enumerate IgA-producing AFCs in the iLP [11] , [13] . Briefly, various concentrations of mononuclear cells were cultured at 37 °C for 4 h in 96-well nitrocellulose membrane plates (Millititer HA; Millipore, Bedford, MA) coated with 1 mg ml −1 OVA and 5 μg ml −1 bovine serum albumin-conjugated phosphorylcholine (Biosearch Technologies, Novato, CA). After vigorous washing of the plates with PBS and PBS containing 0.05% Tween 20, HRP-conjugated goat anti-mouse IgA was added; the plates were then incubated overnight at 4 °C. Spots of AFCs were developed with 2-amino-9-ethylcarbazole (Polysciences, Warrington, PA). The size of each spot was measured with Zeiss KS ELISPOT software (Oberkochen, Germany). In vitro culture CD11b + IgA + or CD11b − IgA + PCs (10 4 cells per well) were purified from the iLP and cultured with 100 ng ml −1 phorbol 12-myristate 13-acetate plus 300 ng ml −1 ionomycin, or 10 μg ml −1 lipopolysaccharide (all from Sigma-Aldrich), for 24 h. For the bacteria uptake assay, fluorescent Staphylococcus aureus was opsonized in accordance with the manufacturer’s protocol (Molecular Probes). Mononuclear cells isolated from the iLP (2 × 10 5 cells) were incubated with 1 × 10 5 opsonized bacteria for 90 min. After being washed, the cells were stained with antibodies for PE-IgA (mA-6E1, 0.5 μg ml −1 , eBioscience) and Pacific Blue CD11b, and the bacterial uptake by each population was examined by flow cytometry. Microarray analysis Microarray analysis was performed as we previously reported [47] . Briefly, CD11b + IgA + and CD11b − IgA + cells were isolated from the iLP, and total RNA was extracted from them with an RNeasy kit (Qiagen, Dusseldorf, Germany). cRNA was hybridized with DNA probes on a GeneChip Mouse Genome 430 2.0 array (Affymetrix), washed and fluorescence-labelled in accordance with the standard amplification protocol developed by Affymetrix. The fluorescence intensity of each probe was taken to represent the raw expression level and was quantified with GeneChip Operating software (Affymetrix). Data obtained from two independent experiments were analysed with GeneSpring 7.3.1 software (Silicon Genetics). All microarray data have been deposited in the National Center for Biotechnology Information Gene Expression Omnibus database ( www.ncbi.nlm.nih.gov/geo/ ) under the accession no. GSE37225 . Statistics Results were compared by a non-parametric Mann–Whitney’s U -test and unpaired t -test (two tailed) (GraphPad Software, San Diego, CA). Accession codes: Microarray data have been deposited in the National Center for Biotechnology Information Gene Expression Omnibus database under series accession code GSE37225 . How to cite this article: Kunisawa, J. et al . Microbe-dependent CD11b + IgA + plasma cells mediate robust early-phase intestinal IgA responses in mice. Nat. Commun. 4:1772 doi: 10.1038/ncomms2718 (2013).